Na+intercalation pseudocapacitance in graphene-coupled titanium oxide enabling ultra-fast sodium storage and long-term cycling Sodium-ion batteries are emerging as a highly promising technology for large-scale energy storage applications. However, it remains a significant challenge to develop an anode with superior long-term cycling stability and high-rate capability. Here we demonstrate that the Na + intercalation pseudocapacitance in TiO 2 /graphene nanocomposites enables high-rate capability and long cycle life in a sodium-ion battery. This hybrid electrode exhibits a specific capacity of above 90 mA h g −1 at 12,000 mA g −1 ( ∼ 36 C). The capacity is highly reversible for more than 4,000 cycles, the longest demonstrated cyclability to date. First-principle calculations demonstrate that the intimate integration of graphene with TiO 2 reduces the diffusion energy barrier, thus enhancing the Na + intercalation pseudocapacitive process. The Na-ion intercalation pseudocapacitance enabled by tailor-deigned nanostructures represents a promising strategy for developing electrode materials with high power density and long cycle life. Over the past few decades, tremendous efforts have been focused on the development of lithium ion batteries (LIBs) used in portable electric devices and electric vehicles because of their high energy density and long cycle life [1] , [2] , [3] , [4] , [5] . Nowadays, the main concerns about LIBs lie in the growing cost and limited resources of lithium. In contrast, sodium ion batteries (SIBs) represent potential alternatives for large-scale energy storage because of low cost and resource abundance [6] , [7] , [8] . Recently, a variety of cathode materials have been investigated for SIBs, for instance, Na 3 V 2 (PO 4 ) 3 (ref. 9 ), P2-Na x VO 2 (ref. 10 ), olivine-type sodium metal phosphates [11] and Prussian blue [12] . For anode materials in SIBs, various carbon materials have been reported because of their relatively high capacity and cyclability [13] , [14] , [15] . Among them, graphite is an intriguing material with different lithium and sodium storage properties (372 mA h g −1 in LIBs, but less than 35 mA h g −1 in SIBs). Intriguingly, Wang and co-workers [14] reported on an expanded graphite that delivered a high capacity of 284 mA h g −1 and long cycle life by expanding the interlayer of graphite from 0.34 to 0.43 nm. Co-intercalation between graphite and diglyme-based electrolyte could also achieve a relatively high capacity of ∼ 90 mA h g −1 and long cycle life [15] . Recent findings have shown that the anode materials for SIBs based on alloy-type (for example, metallic and intermetallic materials [16] , [17] , [18] , [19] ) and conversion-type (for example, sulfides [20] , [21] , [22] , [23] ) exhibited high initial capacity, but suffered from poor cyclability most likely due to the large volume change and the sluggish kinetics. In addition, organic anode materials (for example, Na 2 C 8 H 4 O 4 ) and carboxylate-based materials have been investigated as anode materials for SIBs [24] , [25] , but the electronic conductivity and cyclability still remain the significant challenge. Besides the aforementioned anode candidates, metal oxide materials [26] , especially Ti-based oxide materials were also proposed as anode materials for SIBs. Xiong and co-workers [27] reported the first TiO 2 -based anode for SIBs by using amorphous TiO 2 nanowires grown on a Ti substrate, which delivered a gradually increasing capacity of up to 120 mA h g −1 at 50 mA g −1 . Recently, Myung et al . [28] reported that a thin carbon layer coated on anatase TiO 2 nanorods helped enhance rate capability. They also proposed that the sodiation process of anatase nanorods is an intercalation reaction instead of an alloying reaction. Despite these advances, the long-term cyclability and detailed sodium storage mechanisms still need to be further explored. Another type of TiO 2 , termed TiO 2 -B, has also aroused interest as an anode for SIBs [29] . For insertion-type anodes, the tradeoff between structural stability and capacity should be taken into account. It is highly challenging but desirable to find an effective way to enhance the electrochemistry without sacrificing the stability of the host structure. Recently, pseudocapacitive charge storage that is not a diffusion-controlled process demonstrates superior high-rate performance and reversibility [30] , [31] , [32] , [33] . Previous works by Dunn and co-workers [30] show great promise towards high-rate electrodes in LIBs driven by an intercalation pseudocapacitive mechanism. Inspired by this, it is highly expected to achieve superior rate capability and long cycle life of SIBs by introducing intercalation pseudocapacitive charge storage mechanism in electrodes. As far as we know, there have been several investigations focused on the surface redox reaction pseudocapacitance in a thin-film electrode of SIBs with most of the active material at the surface or subsurface [31] , [34] , rather than the intercalation pseudocapacitance. Here we report a SIB anode material, the graphene-coupled TiO 2 sandwich-like hybrid (referred to as G-TiO 2 ). The G-TiO 2 electrode exhibits a superior rate capability and a super long-term cyclability. We first demonstrated that intercalation pseudocapacitance dominates the charge storage process in the G-TiO 2 SIB anode, which contributes to the excellent rate capability and long-term stability. Furthermore, density functional theory (DFT) calculations were further performed to identify the structural characteristics and the sodiation mechanism of the G-TiO 2 electrode. Morphology and structure of the sandwich-like G-TiO 2 The G-TiO 2 hybrid was prepared by a rapid microwave-assisted in-situ reduction-hydrolysis route using TiCl 3 and graphene oxide (GO) in ethylene glycol as the precursor (the detailed procedure is described in the Methods section). A subsequent heat treatment in air removed the residual organics and improved the crystallinity of the product. The experimental and simulated X-ray diffraction (XRD) patterns of the product with Rietveld refinement are presented in Fig. 1a . The XRD peaks can be indexed to the monoclinic TiO 2 -B phase (JCPDF No. 74–1940) and tetragonal anatase (JCPDF No. 65–5714), respectively. Anatase TiO 2 may originate from the partial transformation of metastable TiO 2 -B under heating treatment [35] , [36] , [37] , [38] . Refinement results quantify a mass percentage of ca. 76.9% for the TiO 2 -B phase (the calculation details are presented in Supplementary Method ), which can be further confirmed by Raman analysis based on the peak areas of Raman spectra ( ∼ 74%, Supplementary Fig. 1 ). The morphology of the product was identified by scanning electron microscopy (SEM) and transmission electron microscopy (TEM). As shown in Fig. 1b , three-dimensional microsheet-connected networks with macropores could be distinctly observed. The SEM image at a higher magnification ( Fig. 1c ) reveals that there are numerous nanosheet arrays on both sides of the graphene sheets, forming a sandwich-like microstructure. The TEM image in Fig. 1d further confirms the unique nanosheet-on-microsheet sandwich-like architecture. Meanwhile, a nanoporous feature could also be observed in Fig. 1d,e , which is further evidenced by the nitrogen adsorption–desorption measurement ( Supplementary Fig. 2 ). Interestingly, numerous tiny nanoclusters ( ∼ 3–5 nm) are also formed on the graphene sheet ( Fig. 1e ). The high-resolution TEM image ( Fig. 1f ) reveals clear lattices with spacings of 0.62 and 0.35 nm, respectively, indicating the existence of both TiO 2 -B and anatase TiO 2 . The carbon content in the G-TiO 2 hybrid is evaluated to be about 10 wt% by thermogravimetry (TG) analysis ( Supplementary Fig. 3 ). 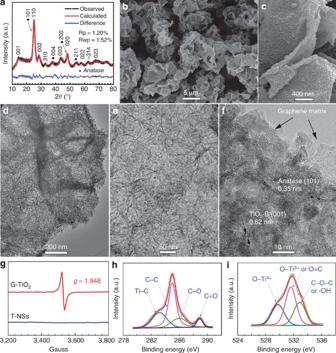Figure 1: Morphology and structure of the G-TiO2hybrid. (a) XRD patterns for the G-TiO2product with Rietveld refinement, quantifying the content of ca 76.9 wt.% for the TiO2-B phase. Calculation details were supplemented inSupplementary Method 1. (b) Low-magnification SEM image for G-TiO2, demonstrating a three-dimensional porous morphology. (c) High-magnification SEM image for G-TiO2, revealing the structural detail of an individual microsheet. (d,e) TEM images for G-TiO2, indicating that tiny nanosheet arrays and nanoparticles co-anchor on the graphene sheet. (f) High-resolution TEM image, clear lattices with spacings of 0.62 and 0.35 nm are assigned to the (001) plane of TiO2-B and (101) plane of anatase, respectively. (g) EPR spectra for the G-TiO2and T-NSs products. (h,i) High-resolution XPS spectra of C 1 s and O 1 s in the G-TiO2product. Figure 1: Morphology and structure of the G-TiO 2 hybrid. ( a ) XRD patterns for the G-TiO 2 product with Rietveld refinement, quantifying the content of ca 76.9 wt.% for the TiO 2 -B phase. Calculation details were supplemented in Supplementary Method 1 . ( b ) Low-magnification SEM image for G-TiO 2 , demonstrating a three-dimensional porous morphology. ( c ) High-magnification SEM image for G-TiO 2 , revealing the structural detail of an individual microsheet. ( d , e ) TEM images for G-TiO 2 , indicating that tiny nanosheet arrays and nanoparticles co-anchor on the graphene sheet. ( f ) High-resolution TEM image, clear lattices with spacings of 0.62 and 0.35 nm are assigned to the (001) plane of TiO 2 -B and (101) plane of anatase, respectively. ( g ) EPR spectra for the G-TiO 2 and T-NSs products. ( h , i ) High-resolution XPS spectra of C 1 s and O 1 s in the G-TiO 2 product. Full size image The surface chemical bonding state of the G-TiO 2 hybrid was determined by electron paramagnetic resonance (EPR) and X-ray photoelectron spectroscopy (XPS). The sample of TiO 2 nanosheets (T-NSs) without GO do not exhibit characteristic EPR response, whereas the G-TiO 2 hybrid presents a distinct EPR signal with a g value of 1.948, indicating the existence of Ti 3+ on the surface of the material ( Fig. 1g ) [39] , [40] . The existence of Ti 3+ was further confirmed by the high-resolution XPS spectra of C 1 s and O 1 s ( Fig 1h,i ). The peaks at 285.0, 286.5 and 288.5 eV are associated with the carbon species from the graphene or the atmosphere. The peak at 283.5 eV suggests the existence of the Ti-C bonds in the G-TiO 2 (ref. 40 ), which is also revealed by the O 1 s peak at 531.5 eV for the O-Ti 3+ bond. The combination of the EPR and XPS results suggests that TiO 2 nanosheets and/or nanoclusters are chemically bonded with the graphene matrix rather than physical adsorption. 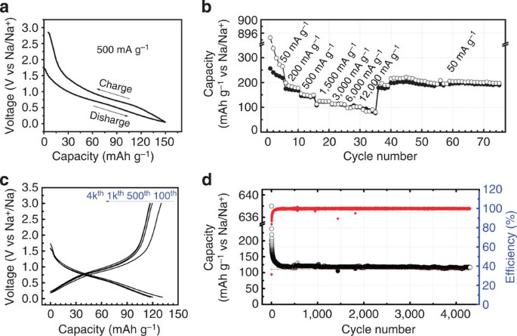Figure 2: Electrochemical performance of the G-TiO2electrode. (a) Galvanostatic cycling profile with a narrow ΔE. (b) Rate performance at various current densities from 50 to 12,000 mA g−1. (c) Charge–discharge profiles from selected cycles of 100th to 4,000th at 500 mA g−1. (d) Long-term cycling performance at a current density of 500 mA g−1(∼2 C). Sodium ion storage performance Figure 2 demonstrates the representative galvanostatic cycling profiles for the G-TiO 2 electrode obtained at 500 mA g −1 . The potential profiles are sloping curves, delivering a discharge capacity of 149 mA h g −1 . Importantly, the polarization between the charge/discharge curves is very small (Δ E = ∼ 0.1 V). Furthermore, the sodium ion storage is mainly below 1.5 V with an average discharging voltage plateau at ∼ 0.8 V, much lower than those in a lithium cell (1.5 V for TiO 2 -B and 1.75 V for anatase TiO 2 ). Further DFT calculations of the voltage profiles based on the sodium intercalation energies in bulk TiO 2 -B with sodium concentrations of x =0.065–0.5 demonstrate an average discharging voltage of ∼ 1.0 V, slightly higher ( ∼ 0.2 V) than the experimental value ( Supplementary Fig. 4 ). Despite the calculation error caused by the overbinding of sodium metal and problems with dispersion term [41] , there are two factors that result in the differences between the experimental and calculated voltages: (i) polarization in the electrode material; (ii) sodiation energetic kinetics differences between nanosized and bulk TiO 2 materials. As polarization is dependent on the current density (namely, higher current densities would lead to bigger polarizations), the difference in the applied current densities of the experimental and calculated data (500 mA h g −1 for the former and infinitely near zero at the equilibrium state for the latter) should be partially responsible for the difference between the two voltages. Previous works reveal that the alkalization potential of nanosized materials could differ from their corresponding bulk materials, due to the alkalization energetic kinetics differences between them [42] . Lower average lithiation potentials in nanosized TiO 2 than bulk TiO 2 materials have been observed in several TiO 2 -Li cells [43] , [44] . Similar effects on the average sodiation potentials are observed in the present work, possibly resulting from the ultrafine nanocrystals in the TiO 2 -graphene hybrid. As a negative electrode, the lower operation voltage in SIBs than in LIBs would lead to a higher energy density of full cells [45] . Meanwhile, the relatively higher sodiation voltage than hard carbon ( ∼ 0.1 V) and Na 2 Ti 3 O 7 (0.3 V) makes the G-TiO 2 much safer and avoids the formation of dendrites upon cycling [46] . Figure 2: Electrochemical performance of the G-TiO 2 electrode. ( a ) Galvanostatic cycling profile with a narrow Δ E . ( b ) Rate performance at various current densities from 50 to 12,000 mA g −1 . ( c ) Charge–discharge profiles from selected cycles of 100th to 4,000th at 500 mA g −1 . ( d ) Long-term cycling performance at a current density of 500 mA g −1 ( ∼ 2 C). Full size image Another attractive property of the chemically bonded G-TiO 2 electrode is the superior rate performance, as presented in Fig. 2b . It can deliver reversible capacities of 265, 187, 149, 125, 114 and 102 mA h g −1 at 50, 200, 500, 1,500, 3,000, and 6,000 mA g −1 , respectively. More excitingly, at an extremely high current density of 12,000 mA g −1 (ca 36 C, assuming 1 C=330 mA g −1 ), a surprisingly high capacity of more than 90 mA h g −1 can still be retained. To the best of our knowledge, this is the best rate capability among all reported Ti-based anode materials as well as the hard carbon and other metal oxides for SIBs [28] , [29] , [47] , [48] . Long-term cyclability is crucial but challenging for rechargeable SIBs, due to the difficulty in the insertion/extraction of the large sodium ions within the host, as well as the side reactions between the electrode and the electrolyte upon long-term cycling. In this regard, we have evaluated the cycling stability of the G-TiO 2 electrode. Figure 2d shows the long-term cycling performance of the G-TiO 2 electrode for over 4,300 cycles at a current rate of 500 mA g −1 . After a slow capacity fading in the initial dozens of cycles, a reversible capacity of 120 mA h g −1 keeps unchanged during the subsequent cycles, indicating a superior long-term cyclability. As far as we know, this is the longest cycle life up to date for both anode and cathode materials for SIBs using nonaqueous electrolytes [7] , [8] , [9] , [10] , [11] , [12] , [13] , [14] , [15] , [16] , [17] , [18] , [19] , [20] , [21] , [22] , [23] , [24] , [25] , [26] , [27] , [28] , [29] , [32] , [33] , [34] , [47] , [48] . We should also note that the Coulombic efficiency increased gradually up to 91.8% during the initial cycles. The irreversible capacity loss during initial cycles may result from the formation of a solid electrolyte interface film (caused by reactions between the surface –OH groups of titania and the carbonate-based electrolyte) [49] , and the irreversible trapping of sodium ions at active sites of the graphene matrix [50] . It was reported that a pre-sodiation or chemical treatment could mitigate the irreversible capacity loss [28] , [49] . By replacing polyvinylidene fluoride (PVDF) with sodium polyacrylate (PAA-Na) as the binder or pretreating the G-TiO 2 hybrid material with butyl lithium, the initial Coulombic efficiency can be enhanced from 31.4% to ∼ 57.0% and 58.4%, respectively ( Supplementary Fig. 5 ). Furthermore, a combined use of the PAA-Na binder and pretreatment leads to a much higher initial Coulombic efficiency, up to 80.6% ( Supplementary Fig. 5 and Supplementary Table 1 ). Our preliminary results demonstrate that the irreversible capacity loss of the G-TiO 2 electrode upon cycling could be further reduced by optimizing the binder or the electrode surface. Figure 2c shows the galvanostatic charge–discharge profiles for the 100th, 500th, 1,000th, and 4,000th cycles. They possess an average voltage plateau at ∼ 0.8 V, revealing the structural stability and the high reversibility of the insertion/extraction of sodium ions within the host material. When the potential window is narrowed to 0.05−1.5 V, there is no significant change of the voltage curves ( Supplementary Fig. 6 ), despite a slightly decrease in discharge capacity ( ∼ 110 mA h g −1 , ca 10 mA h g −1 lower than the former). For comparison, we also explored the electrochemical performances of two pristine TiO 2 nanostructures: (i) T-NSs that were prepared at the similar conditions for G-TiO 2 except using GO and (ii) TiO 2 nanobelts (T-NBs) obtained according to ref. 51 . It was found that the electrode made of pristine TiO 2 nanosheets exhibited a much lower capacity of ∼ 70 mA h g −1 , corresponding to 0.21 Na insertion into a formula of TiO 2 ( Supplementary Fig. 7a ). Its capacity decayed drastically to below 20 mA h g −1 after 50 cycles. Similarly, the performance of the T-NBs electrode was also much worse than that of G-TiO 2 ( Supplementary Fig. 7b ). The synergistic effect from nanostructuring and hybridization might contribute to the substantial enhancement of the G-TiO 2 electrode, where the electronic/ionic conductivity is improved, and high reversibility of chemically bonded G-TiO 2 is achieved. Furthermore, STEM and HR-TEM images, energy dispersive X-ray elemental mappings and selected-area electron diffraction patterns confirm that the microstructure of the strongly coupled G-TiO 2 hybrid is well maintained even after 4,300 discharge/charge cycles ( Supplementary Fig. 8 ). More importantly, the unique graphene-TiO 2 interface in the G-TiO 2 hybrid provides a more feasible pathway for Na + insertion/extraction and prompts an intercalation pseudocapacitive behaviour of Na + in the G-TiO 2 electrode. It is highly beneficial to the fast transport of Na + , thus leading to superior rate capability and long cycle life. Kinetics analysis Cyclic voltammetry (CV) has been proven to be a powerful technique to evaluate the electrochemical kinetics of electrode materials towards Li + or Na + (refs 30 , 31 , 32 , 33 ). Here, kinetic analysis based on CV analysis was carried out to gain further insight into the electrochemistry of the G-TiO 2 /Na cell. 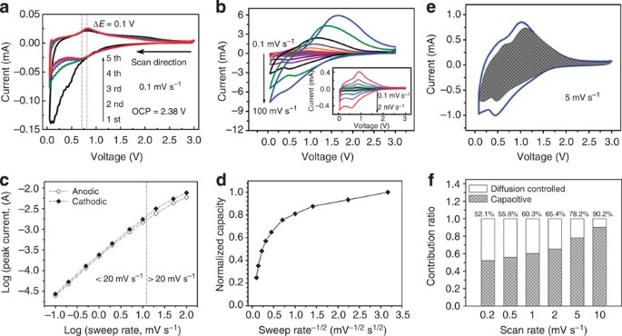Figure 3: Kinetics analysis of the electrochemical behaviour towards Na+for the G-TiO2electrode. (a) CV curves from 1st to 5th cycles at a scan rate of 0.1 mV s−1. The open circuit potential (OCP) is ca 2.38 V. (b) CV curves at various scan rates, from 0.1 to 100 mV s−1. (c) Determination of theb-value using the relationship between peak current and scan rate. (d) Capacity versus scan rate−1/2. (e) Separation of the capacitive and diffusion currents in G-TiO2at a scan rate of 5 mV s−1. (f) Contribution ratio of the capacitive and diffusion-controlled charge versus scan rate. Figure 3a displays the typical CV curves for the G-TiO 2 electrode during initial five cycles at a scan rate of 0.1 mV s −1 . A pair of broad cathodic/anodic peaks are located at ∼ 0.75/0.85 V with a small voltage offset of 0.1 V, which agree well with the galvanostatic cycling profile. Meanwhile, the CV curves from the 3rd to the 5th cycle are overlapped, showing an excellent reversibility of the G-TiO 2 electrode. The CV curves at various scan rates from 0.1 to 100 mV s −1 display similar shapes with broad peaks during both cathodic and anodic processes. It is interesting to note that the small peak separations ( ∼ 0.1 V) are nearly identical if the scan rate increases from 0.1 to 2 mV s −1 (inset of Fig. 3b and Supplementary Fig. 9 ), demonstrating small polarization at high rates. According to the relationship between the measured current ( i ) and the scan rate ( v ) [52] : Figure 3: Kinetics analysis of the electrochemical behaviour towards Na + for the G-TiO 2 electrode. ( a ) CV curves from 1st to 5th cycles at a scan rate of 0.1 mV s −1 . The open circuit potential (OCP) is ca 2.38 V. ( b ) CV curves at various scan rates, from 0.1 to 100 mV s −1 . ( c ) Determination of the b -value using the relationship between peak current and scan rate. ( d ) Capacity versus scan rate −1/2 . ( e ) Separation of the capacitive and diffusion currents in G-TiO 2 at a scan rate of 5 mV s −1 . ( f ) Contribution ratio of the capacitive and diffusion-controlled charge versus scan rate. Full size image the b -value can be determined by the slope of the log( v )–log( i ) plots. In particular, the b -value of 0.5 indicates a total diffusion-controlled behaviour, whereas 1.0 represents a capacitive process. The log( v )–log( i ) plots for the G-TiO 2 electrode is shown in Fig. 3c . The b -value of 0.94 for both cathodic and anodic peaks can be quantified at scan rates from 0.1 to 10 mV s −1 , suggesting the kinetics of capacitive characteristics. A decrease of slope takes place at scan rates above 10 mV s −1 , reflecting a decrease of b -value from 0.94 to 0.56 for both cathodic and anodic peaks. Similar observations were reported on a T -Nb 2 O 5 /Li cell by Dunn et al . [30] The limitation to the rate capability should be attributed to an increase of the ohmic contribution and/or diffusion constrains upon an ultra-fast scan rate. The b -value of 0.56 close to 0.5 evidences the limitation of the slow diffusion. The plot of capacity versus v −1/2 demonstrates that the capacity does not vary significantly as the scan rate increases in the range of 0.1–2 mV s −1 ( Fig. 3d ). This indicates that capacitive contributions are independent of the scan rate. In contrast, the linear decrease of capacity upon the increase of scan rate in the region of >10 mV s −1 reflects a rate-limited diffusion process. The total capacitive contribution at a certain scan rate could be quantified on the base of separating the specific contribution from the capacitive and diffusion-controlled charge at a fixed voltage. As shown in Fig. 3e , the diffusion-controlled charge is mainly generated at around the peak voltage, indicating that the diffusion process is feasible at this region and corresponds to a redox reaction between Ti 4+ /Ti 3+ (ref. 44 ). Based on the quantification, 78.2% of the total charge (therefore, the capacity) is capacitive at a scan rate of 5 mV s −1 . Contribution ratios between the two different processes at other scan rates were also quantified. The quantified results ( Fig. 3f ) show that the capacitive capacity is improved gradually with increasing the scan rate, and finally reaches a maximum value of 90.2% at 10 mV s −1 . The Na + intercalation pseudocapacitive behaviour of the G-TiO 2 hybrid is attributed to the unique chemically bonded hybrid structure that provides a more feasible channel for Na + insertion/extraction in the graphene–TiO 2 interface. First-principle calculations were performed to obtain further insight into the Na + dynamics in the G-TiO 2 hybrid and to testify this hypothesis. As the main phase of the hybrid is TiO 2 -B, only TiO 2 -B was taken into account in the first-principle calculations. From the voltage profiles ( Fig. 2e ), it is observed that the voltage drops monotonically from 1.15 V down to 0.05 V. This suggests a solid-solution reaction of sodium with TiO 2 at an average voltage of ∼ 0.8 V. The calculated voltage profiles show a similar dropping trend, despite the slightly higher values for the calculated voltages ( Supplementary Fig. 4 ). To gain further insight into the sodiation dynamics, sodium-diffusion barriers of various trajectories were also investigated by first-principle calculations. In bulk TiO 2 -B, three typical sodium-diffusion paths were considered, as presented in Supplementary Fig. 10 . The energy barriers for path i, ii and iii were 3.0, 4.9 and 2.2 eV, respectively, which are similar to the previous report on a TiO 2 -B-Li battery [41] . It is reasonable that the energy barriers for sodium insertion into the TiO 2 -B host are higher than that of lithiation, considering the bigger radius of Na + . It means that path i along the [001] direction and path iii along the [010] direction are more accessible for Na + diffusion than path ii ([100] direction). Interestingly, much more feasible paths could be formed at the fully bonded graphene–TiO 2 -B interface in the hybrid ( Supplementary Fig. 11 ). The energy barriers for path iii are reduced to be 1.5 eV. Considering the existence of surface defects in the TiO 2 nanocrystals, surface –OH groups [49] , and the mismatching between TiO 2 -B and graphene lattices, surface oxygen atoms cannot be entirely bonded with the carbon atoms of graphene. The dominated situation should be the partially bonded model, where a part of surface O atoms would be passivated by a neighbouring surface O atom (Ti−O surf. −O surf. −Ti) or surface –OH groups (Ti−O surf. −Η), rather than the formation of Ti−O−C bonds, to achieve a lower total energy of the system ( Supplementary Fig. 12 ). Owing to the reduction of bonded surface oxygen atoms, the restriction to graphene by the TiO 2 -B nanocrystals becomes weaker, resulting in the slightly bending of graphene plate ( Fig. 4 ). Consequently, the tunnel along the [010] direction will be more open and feasible for sodium transport, giving rise to a much lower activation energy barrier of ∼ 0.2 eV ( Fig. 4 , unbounded surface O atoms reconstitute to form Ti−O surf. −O surf. −Ti) or 0.45 eV ( Supplementary Fig. 13 , unbounded surface O atoms were passivated by the –OH groups). The isolated sodium diffusion should be much different from a certain concentration region in this system. In fact, the pervious results on the lithium diffusion in anatase TiO 2 with the Li concentration of 10–50% revealed that an increase in Li concentration resulted in a decrease in effective barrier (namely, it would be more diffusive with an increased Li concentration) [53] . It is much likely to occur in our system that the diffusion of sodium ions will be more feasible upon increasing sodium concentration. These calculation results agree well with the experimental results presented above. 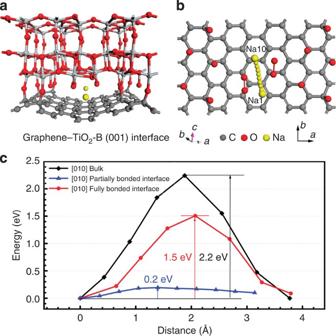Figure 4: Na diffusion in the partially bonded graphene–TiO2-B (001) interface. (a) Illustration of the partially bonded graphene–TiO2-B (001) interface. (b) Top-view ofa, illustrating the Na diffusion path along the [010] direction from Na1 to Na10 sites. (c) Migration activation energy of the Na+ion diffusing along the [010] direction in bulk TiO2-B, fully bonded and partially bonded graphene–TiO2-B (001) interface calculated with DFT. Figure 4: Na diffusion in the partially bonded graphene–TiO 2 -B (001) interface. ( a ) Illustration of the partially bonded graphene–TiO 2 -B (001) interface. ( b ) Top-view of a , illustrating the Na diffusion path along the [010] direction from Na1 to Na10 sites. ( c ) Migration activation energy of the Na + ion diffusing along the [010] direction in bulk TiO 2 -B, fully bonded and partially bonded graphene–TiO 2 -B (001) interface calculated with DFT. Full size image In summary, the chemically bonded graphene-TiO 2 hybrid demonstrates a reversible capacity of 265 mA h g −1 at 50 mA g −1 and more than 90 mA h g −1 at 12,000 mA g −1 ( ∼ 36 C), displaying the best rate capability compared with the ever reported Ti-based anodes for SIBs. More encouragingly, the hybrid electrode shows an ultra-long cycling life as demonstrated by over 4,300 cycles, representing the best cyclability among all ever reported SIBs using nonaqueous electrolytes. Kinetics analysis reveals an interesting Na + intercalation pseudocapacitive behaviour in the G-TiO 2 sodium cell and a high contribution of capacitive charge. This pseudocapacitive behaviour is highly beneficial to fast charge storage and long-term cyclability. Further sodiation dynamics analysis based on first-principle calculations shows that the hybridization of graphene with TiO 2 nanocrystals provides a more feasible channel at the graphene–TiO 2 interface for sodium intercalation/deintercalation with a much lower energy barrier. Our findings will open up new opportunities for developing electrode materials of SIBs and hold great promise for the development of long-life SIBs for next-generation large-scale energy storage applications. Materials synthesis The G-TiO 2 hybrid was prepared by a microwave-assisted reduction-hydrolysis route. The mixture of TiCl 3 (1 ml, 15 wt% in dilute hydrochloric acid solution), ethylene glycol (15 ml, anhydrous) and GO (2 ml, 13 mg ml −1 , prepared via a modified Hummers method [54] ) was sealed in a glass vessel and treated in a microwave synthesizer (2.45 GHz, 300 W, Discover S-Class, CEM) at 155 °C for 30 min. The black product was collected by centrifugation, and washed with DI water and ethanol for five times. After dry at 80 °C overnight, the black powder was heated at 350 °C for 4 h in air to remove the residual organics, and finally the G-TiO 2 product was obtained. In a control experiment, the T-NSs product was prepared by a similar method to that of G-TiO 2 except the use of GO. The T-NBs product was prepared according to the previous report [51] . For the pretreatment procedure, the materials treated with bultyl lithium were obtained by dispersing G-TiO 2 powder (128 mg) in 25 ml of hexane and adding dropwise into a suspension of bultyl lithium hexane solution (0.25 ml, 1.6 M). After stirred for 3 h, the suspension was filtered and washed with hexane, and dried under vacuum at 60 °C for 8 h. Materials characterization The morphology and structure of the products were investigated by SEM (SIRION200), TEM, XRD (PANalytical B.V.) and XPS (VG MultiLab 2000 system with a monochromatic A1 Kα X-ray source, Thermo VG Scientific). TG analysis was carried out in air atmosphere from 40 to 750 °C at a heating rate of 10 °C min −1 . Nitrogen adsorption and desorption isotherms and pore size distribution were collected at 77 K using a Micromeritics ASPA 2020 analyzer. EPR measurements were performed on a Bruker EMX spectrometer equipped with a cylindrical cavity operating at a 100 kHz field modulation at 77 K. Raman spectra were obtained on a Renishaw Invia spectrometer with an Ar + laser of 514.5 nm at room temperature. Electrochemical measurements The working electrodes were prepared by mixing 70 wt% active material, 20 wt% super P and 10 wt% PVDF dissolved in N -methyl-2-pyrrolidone (for comparison, PVDF was also replaced by PAA-Na to mitigate the irreversible capacity loss), and then coated onto a Cu foil and dried at 80 °C for 24 h before testing. The mass loading of the active material is about 2.5 mg cm −2 . The testing cell contains the working electrode, sodium metal as the counter and reference electrode, glass fibre membrane (GF/D, Whatman) as the separator and 1 M NaClO 4 in a mixture of ethylene carbonate and propylene carbonate (2:1 by volume) as the electrolyte. Galvanostatic charge–discharge tests were carried out on a Land Battery Measurement System (Land) at various current densities with a cutoff potential window of 0.05–3 V at room temperature. CV measurements at various scan rates from 0.1 to 100 mV s −1 were carried out on a PARSTAT 2273 potentiostat. DFT calculations First-principle calculations were performed using the Vienna Ab Initio Simulation Package [55] within the projector augmented-wave approach. The generalized gradient approximation (GGA) exchange-correlation function developed by Perdew, Burke and Ernzerhof [56] was used and the cutoff of the kinetic energy was set to 400 eV for all calculations. As the Ti-based oxides are strongly correlated electron systems, the DFT+U method was used with the Dudarev approach [57] implemented in Vienna Ab Initio Simulation Package, where U is the on-site Coulomb parameter to calculate the average voltages of Na intercalating into TiO 2 -B. On the other hand, the standard GGA functional is used instead of the GGA+U functional for the diffusion barrier calculations to avoid the mixing charge transfer barrier of alkali atoms hoping overestimated by the GGA+U method [45] . The k-points were sampled on a Γ-centred Monkhorst-Pack grid of 4 × 8 × 6 for the unit cell and the geometry was allowed to relax until Hellmann–Feynman force on each atom was less than 0.05 eV Å −1 . The minimum energy paths and activation barriers of Na diffusion along different channels were calculated by the climbing nudged elastic band method [58] for the bulk TiO 2 -B and TiO 2 -B–graphene interface. For Na diffusion in bulk TiO 2 -B, a 1 × 2 × 1 supercell was used to minimize the interaction between the periodic images. To model the TiO 2 -B–graphene interface, a 1 × 2 supercell of TiO 2 -B (001) slab square lattice (12.29 × 7.55 Å) with thickness of about 10 Å was constructed to match with the graphene square lattice with a 3 × 3 supercell (12.78 × 7.38 Å), including 36 C atoms. The lattice mismatch in each direction was less than 5%. For more precise results, a vacuum thickness of 20 Å was set along c axis for the TiO 2 -B–graphene to avoid the interaction between neighbouring images. How to cite this article : Chen, C. et al . Na+ intercalation pseudocapacitance in graphene-coupled titanium oxide enabling ultra-fast sodium storage and long-term cycling. Nat. Commun . 6:6929 doi: 10.1038/ncomms7929 (2015).